Endogenous Wnt signalling in human embryonic stem cells generates an equilibrium of distinct lineage-specified progenitors The pluripotent nature of human embryonic stem cells (hESCs) makes them convenient for deriving therapeutically relevant cells. Here we show using Wnt reporter hESC lines that the cells are heterogeneous with respect to endogenous Wnt signalling activity. Moreover, the level of Wnt signalling activity in individual cells correlates with differences in clonogenic potential and lineage-specific differentiation propensity. The addition of Wnt protein or, conversely, a small-molecule Wnt inhibitor (IWP2) reduces heterogeneity, allowing stable expansion of Wnt high or Wnt low hESC populations, respectively. On differentiation, the Wnt high hESCs predominantly form endodermal and cardiac cells, whereas the Wnt low hESCs generate primarily neuroectodermal cells. Thus, heterogeneity with respect to endogenous Wnt signalling underlies much of the inefficiency in directing hESCs towards specific cell types. The relatively uniform differentiation potential of the Wnt high and Wnt low hESCs leads to faster and more efficient derivation of targeted cell types from these populations. The pluripotent nature of human embryonic stem cells (hESCs) makes them a convenient in vitro model for studying aspects of early development and a common starting point for deriving numerous therapeutically relevant cells. Although it is often assumed that hESCs exist as a homogenous population of pluripotent cells, recent studies suggest hESC cultures contain significant heterogeneity. For example, SSEA-3 expression level distinguishes two populations of undifferentiated hESCs with different proliferation rates, clonogenic potential and OCT4 protein levels [1] . Even among hESCs with uniformly high OCT4, Nanog and SSEA-3 expression, distinct subpopulations with lineage-specific epiblast stem cells surface markers and differentiation propensities have been found [2] . Similar heterogeneity is found in mouse embryonic stem cells [3] and epiblast stem cells (EpiSCs) [4] . In all of these cases, clonally isolated subpopulations rapidly re-establish the other populations, suggesting efficient maintenance of equilibrium among the different subpopulations. This persistent heterogeneity within hESC cultures makes it difficult to rigorously establish the roles of specific signalling molecules, and this may underlie the poor efficiency of directed differentiation towards specific cell types [5] , [6] . Thus, the ability to stably maintain homogenous populations of pluripotent hESCs would greatly improve their utility. Wnt signalling has been widely implicated in hESC biology, but there is disagreement about whether Wnt signalling promotes self-renewal or differentiation [7] , [8] , [9] , [10] , [11] , [12] , [13] . Here we used Wnt reporter hESC lines, to establish that the cells are heterogeneous with respect to endogenous Wnt signalling activity. By manipulating Wnt signals, we reduced heterogeneity leading to a more efficient derivation of targeted cell types from hESCs. Wnt reporter hESC lines are heterogeneous To monitor Wnt pathway activity in living cells, we generated clonal H9 hESC lines carrying a stably integrated TCF-GFP reporter [14] ( Fig. 1a ). We observed a range of TCF-GFP expression patterns, from colonies with no detectable expression to colonies with expression in cells at the periphery and expression throughout. Stimulating Wnt signalling with purified Wnt3a protein or CHIR99021, a small-molecule GSK3β-inhibitor, resulted in uniformly high green fluorescent protein (GFP) expression ( Fig. 1b ). Conversely, inhibiting endogenous Wnt signalling with IWP2-lowered GFP expression ( Fig. 1b ), confirming the fidelity of our reporter lines. Our ability to detect endogenous Wnt pathway activity in hESCs differs from previous reports using transient transfections [8] , [9] , reflecting the importance of using genomically integrated, non-silenced, reporters. 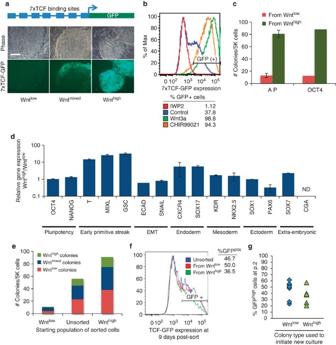Figure 1: Endogenous Wnt signalling reveals distinct subpopulations of hESCs. Analysis of transgenic 7xTCF-GFP hESCs in standard self-renewing conditions. (a) TCF-GFP expression pattern in live hESC colonies. Scale bar, 200 μm. (b) FACS analysis of TCF-GFP expression in live cells after 4 days of IWP2, Wnt3a or CHIR99021 treatment. Pre-gated for live, non-mouse cells. (c) Quantitative Clonogenic Potential Assay. Double FACS-sorted populations of TCF-GFPhighand TCF-GFPlowcells were plated as single cells in standard hESC. Clonogenic potential was determined by counting the number of alkaline phosphatase (AP)-positive (left) and OCT4-positive (right) colonies 7 days after plating. Error bars show the range of two biological replicates and are representative of three independent experiments. (d) Gene expression analysis in double FACS-sorted populations of >99.5% purity. The ratio of glyceraldehyde 3-phosphate dehydrogenase-normalized gene expression level in TCF-GFPhighhESCs divided by TCF-GFPlowhESCs is shown. ND, not detectable. ±s.d of three biological replicates and are representative of two independent experiments. (e) GFP expression pattern of live colonies derived from plating single cells of >99.5% pure populations at clonal density (500 cells per cm2) in standard self-renewing conditions. The starting populations are indicated on thexaxis, examples of the three GFP expression patterns counted are shown ina. (f) FACS analysis of GFP expression in hESC cultures 9 days after plating single cells from the indicated population of sorted cells. %GFPposis based on live, non-mouse cells. (g) FACS analysis of GFP expression in hESC passage 2 cultures initiated from single colonies that were entirely GFPlowor GFPhigh. %GFPposis based on live, non-mouse cells. Figure 1: Endogenous Wnt signalling reveals distinct subpopulations of hESCs. Analysis of transgenic 7xTCF-GFP hESCs in standard self-renewing conditions. ( a ) TCF-GFP expression pattern in live hESC colonies. Scale bar, 200 μm. ( b ) FACS analysis of TCF-GFP expression in live cells after 4 days of IWP2, Wnt3a or CHIR99021 treatment. Pre-gated for live, non-mouse cells. ( c ) Quantitative Clonogenic Potential Assay. Double FACS-sorted populations of TCF-GFP high and TCF-GFP low cells were plated as single cells in standard hESC. Clonogenic potential was determined by counting the number of alkaline phosphatase (AP)-positive (left) and OCT4-positive (right) colonies 7 days after plating. Error bars show the range of two biological replicates and are representative of three independent experiments. ( d ) Gene expression analysis in double FACS-sorted populations of >99.5% purity. The ratio of glyceraldehyde 3-phosphate dehydrogenase-normalized gene expression level in TCF-GFP high hESCs divided by TCF-GFP low hESCs is shown. ND, not detectable. ±s.d of three biological replicates and are representative of two independent experiments. ( e ) GFP expression pattern of live colonies derived from plating single cells of >99.5% pure populations at clonal density (500 cells per cm 2 ) in standard self-renewing conditions. The starting populations are indicated on the x axis, examples of the three GFP expression patterns counted are shown in a . ( f ) FACS analysis of GFP expression in hESC cultures 9 days after plating single cells from the indicated population of sorted cells. %GFP pos is based on live, non-mouse cells. ( g ) FACS analysis of GFP expression in hESC passage 2 cultures initiated from single colonies that were entirely GFP low or GFP high . %GFP pos is based on live, non-mouse cells. Full size image hESCs with various levels of Wnt activity differed from each other in several respects. We measured the self-renewal potential of individual Wnt high or Wnt low cells using a quantitative clonogenic potential assay [1] , [2] . hESCs were sorted into populations of greater than 99.5% pure Wnt high or Wnt low hESCs using two rounds of fluorescence-activated cell sorting (FACS; Supplementary Fig. S1A ). Wnt high single cells formed more than five times as many alkaline phosphatase (AP)-positive and OCT4-positive pluripotent colonies as Wnt low cells ( Fig. 1c ), despite similar expression of OCT4, SSEA-4 and TRA-1-60 in both starting populations ( Supplementary Fig. S1B–D ). By measuring gene expression in >99.5% pure populations, we found that Wnt high hESCs expressed more than tenfold higher levels of primitive streak/mesoderm markers Brachyury, Mixl1 and Goosecoid, as well as fourfold higher levels of endodermal markers CXCR4 and Sox17 relative to Wnt low hESCs ( Fig. 1d ). In contrast, the neuroectodermal marker Pax6 was higher in Wnt low hESCs. Markers of extra-embryonic endoderm (SOX7) and trophectoderm (CGA) were unchanged or undetectable in either population. Thus, even among cells with similar expression of pluripotency markers, hESCs are heterogeneous, and cells with different clonogenic potential and epigenetic status can be prospectively identified by monitoring Wnt pathway activity. The enhanced clonogenic potential of Wnt high hESCs did not correlate with elevated expression of pluripotency markers; therefore, we tested whether Wnt signalling could also affect proliferation or survival of hESCs. We found only a very small difference in the percentage of proliferating cells in the Wnt high population of pluripotent cells compared with Wnt low pluripotent cells ( Fig. 2a,b ). Likewise, addition of purified Wnt3a to hESCs did not significantly alter the proliferation of pluripotent cells ( Fig. 2c ). More significantly, we found that Wnt signalling promoted survival of hESCs. When the number of viable hESCs was counted one day after passage as single cells, cultures treated with purified Wnt3a protein for 24 h before passage contained 20% more viable cells ( Fig. 2d ). This effect is likely due to Wnt-mediated inhibition of apoptosis, as overexpression of the apoptosis inhibitor BCL-2 phenocopied the effect of Wnt signalling on hESC clonogenicity ( Fig. 2e ). BCL-2 overexpression was largely epistatic to addition of Wnt protein, supporting the interpretation that Wnt promotes survival of hESCs by inhibiting apoptosis. These data explain how Wnt signalling can simultaneously enhance clonogenicity of hESCs, even though pluripotency markers are not affected and expression of differentiation markers is moderately increased. 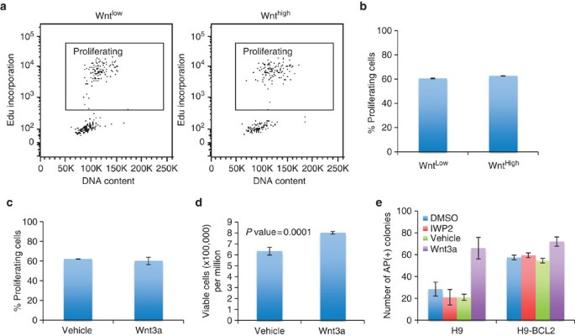Figure 2: Role of Wnt signalling in proliferation and survival. (a) FACS analysis of TCF-GFP hESCs grown in standard hESC conditions showing the number of proliferating (EdU-positive) cells in log-phase cultures (boxed cells). Cells were pre-gated for OCT4-positive non-mouse cells single cells, and separated into either TCFlow(left panel) or TCFhigh(right panel) populations. (b) The percentage of proliferating OCT4-positive cells in TCFlowand TCFhighpopulations inawas averaged across two independent experiments±range. (c) The percentage of proliferating OCT4-positive hESCs after 3 days of treatment with Wnt3a or vehicle was measured as inaandb. The average from two independent experiments is shown. (d) Log-phase hESCs were treated with IWP2 or Wnt3a for 24 h, digested to single cells, counted and plated at 200,000 cells per cm2. The number of viable attached cells still present 24 h after passage was measured. The average number of cells in four replicates of two independent experiments is shown. TheP-value is calculated from a two-tailed equal varianceT-test. (e) Identical numbers of H9 or H9-BCL2 hESCs were plated in standard hESC media on Matrigel in the presence of dimethyl sulfoxide (DMSO; control for IWP2), IWP2, vehicle (control for Wnt3a) or Wnt3a. The number of AP-positive colonies was counted 6 days later. The average of three replicates in a single experiment are shown, ±s.d. Figure 2: Role of Wnt signalling in proliferation and survival. ( a ) FACS analysis of TCF-GFP hESCs grown in standard hESC conditions showing the number of proliferating (EdU-positive) cells in log-phase cultures (boxed cells). Cells were pre-gated for OCT4-positive non-mouse cells single cells, and separated into either TCF low (left panel) or TCF high (right panel) populations. ( b ) The percentage of proliferating OCT4-positive cells in TCF low and TCF high populations in a was averaged across two independent experiments±range. ( c ) The percentage of proliferating OCT4-positive hESCs after 3 days of treatment with Wnt3a or vehicle was measured as in a and b . The average from two independent experiments is shown. ( d ) Log-phase hESCs were treated with IWP2 or Wnt3a for 24 h, digested to single cells, counted and plated at 200,000 cells per cm 2 . The number of viable attached cells still present 24 h after passage was measured. The average number of cells in four replicates of two independent experiments is shown. The P -value is calculated from a two-tailed equal variance T -test. ( e ) Identical numbers of H9 or H9-BCL2 hESCs were plated in standard hESC media on Matrigel in the presence of dimethyl sulfoxide (DMSO; control for IWP2), IWP2, vehicle (control for Wnt3a) or Wnt3a. The number of AP-positive colonies was counted 6 days later. The average of three replicates in a single experiment are shown, ±s.d. Full size image When the sorted populations of Wnt low and Wnt high cells were plated in self-renewing conditions, the heterogeneity was re-established within a single passage ( Fig. 1e,f ). We also initiated new cultures from single colonies that were homogenously GFP negative (Wnt low colonies) or homogenously GFP positive (Wnt high colonies). All of the colonies picked (9/9 GFP low and 6/6 GFP high ) re-established new cultures that contained each of the three colony types shown in Fig. 1a , and FACS analysis showed that all of the clonal cultures now contained a mixture of Wnt low and Wnt high cells ( Fig. 1g ). Culture conditions influence Wnt effects on cells The rapid re-establishment of heterogenous cultures prompted us to attempt to derive more stable homogenous populations by including purified Wnt3a protein or IWP2 in the cultures. Although these experiments were successful, we found that the phenotype of Wnt high hESCs depended on the conditions, in particular, the medium used for cell growth. To more fully understand how growth media altered the Wnt phenotypes, we used three different hESC culture systems. In addition to the 'Standard hESC' conditions used above (feeder cells+serum replacement), we used two defined culture media, N2B27 and mTeSR1, both of which use Matrigel in lieu of feeder cells [15] , [16] . In all media, Wnt3a protein, IWP2 and CHIR99021 induced the expected changes in TCF-GFP reporter expression ( Supplementary Fig. S2A,B ), except that CHIR99021 was less effective in mTeSR1. In terms of effects on hESC behaviour, Wnt signalling influenced cells differently in defined media compared with standard hESC medium. Wnt3a enhanced self-renewal in standard hESC conditions, as indicated by faster accumulation of AP-positive colonies in Wnt3a-treated conditions relative to control buffer (Veh), similar to previous observations [12] . However, Wnt protein caused rapid differentiation in both N2B27 and mTeSR1 ( Fig. 3a,b ). The loss of pluripotent colonies in defined media was accompanied by an increase in total cell number, suggesting that the cells differentiated rather than died ( Fig. 3c ). Differentiation was confirmed by loss of OCT4 expression and gain of Brachyury and GATA4 expression in defined media ( Fig. 3d ). The Wnt inhibitor IWP2 modestly reduced the number of AP+ colonies, roughly proportional to total cell number on standard hESC media, but had little effect in defined media on the number of AP+ colonies or OCT4 staining ( Supplementary Fig. S2C–F ). The overall cell number was reduced after three passages in N2B27 media, possibly due to IWP2 inhibiting secretion of other Wnt proteins required for optimal proliferation on this media ( Supplementary Fig. S2F ). Overall, Wnt signalling promoted expansion of undifferentiated hESCs in standard medium and rapid differentiation of hESCs in defined media. 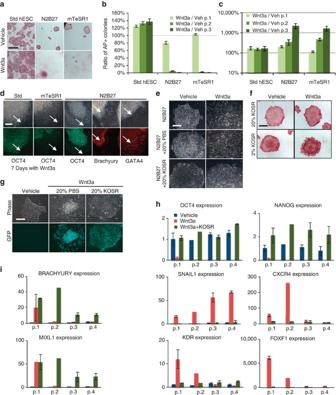Figure 3: Serum replacement blocks Wnt-mediated differentiation. (a) Alkaline phosphatase (AP) staining of cells grown in 'standard (std)', 'N2B27' and 'mTeSR1' media for three passages in the continuous presence of Wnt3a protein or control buffer (vehicle). Scale bar, 2 mm. (b) Quantification of Wnt-mediated changes in self-renewal during passage as clumps. The number of AP+ colonies was determined after each passage. The ratio of cumulative number of AP+ colonies in Wnt3a-treated cultures divided by AP+ colonies in vehicle-treated cultures is shown for each passage in each media. 100% represents an equal number of AP+ colonies in Wnt3a- and vehicle (Veh)-treated cultures. The average ±s.d. of three biological replicates is shown, and is representative of two independent experiments. (c) Quantification of Wnt-mediated changes in total cell number during passage as clumps. The ratio of cumulative cell number in Wnt3a-treated cultures divided vehicle-treated cultures is shown on a log scale. The average ±s.d. of three biological replicates is shown, and is representative of two independent experiments. (d) Phase-contrast and OCT4, Brachyury and GATA4 immunofluorescence images of cells treated with Wnt3a for 7 days in standard hESC media, N2B27 or mTeSR1. Scale bar, 200 μm. (e) Phase-contrast images of hESCs treated for 4 days with Wnt3a in N2B27 media alone, or the same supplemented with 20% PBS or 20% knockout serum replacement (KOSR). Scale bar, 200 μm. (f) AP staining of hESC treated for 3 days with Wnt3a in standard hESC media, or the same media in which the KOSR concentration was reduced to 2%. Scale bar, 200 μm. (g) Phase contrast and GFP fluorescence in live colonies after 5 days of growth on N2B27 in the presence of vehicle, 20% PBS or 20% KOSR. Scale bar, 200 μm. (h,i) Gene expression analysis in cells grown in N2B27 plus the indicated combination of vehicle, Wnt3a and KOSR for four passages. Values were normalized to glyceraldehyde 3-phosphate dehydrogenase, and are expressed relative to vehicle-treated cells at passage 1. The average and range of two biological replicates is shown. Figure 3: Serum replacement blocks Wnt-mediated differentiation. ( a ) Alkaline phosphatase (AP) staining of cells grown in 'standard (std)', 'N2B27' and 'mTeSR1' media for three passages in the continuous presence of Wnt3a protein or control buffer (vehicle). Scale bar, 2 mm. ( b ) Quantification of Wnt-mediated changes in self-renewal during passage as clumps. The number of AP+ colonies was determined after each passage. The ratio of cumulative number of AP+ colonies in Wnt3a-treated cultures divided by AP+ colonies in vehicle-treated cultures is shown for each passage in each media. 100% represents an equal number of AP+ colonies in Wnt3a- and vehicle (Veh)-treated cultures. The average ±s.d. of three biological replicates is shown, and is representative of two independent experiments. ( c ) Quantification of Wnt-mediated changes in total cell number during passage as clumps. The ratio of cumulative cell number in Wnt3a-treated cultures divided vehicle-treated cultures is shown on a log scale. The average ±s.d. of three biological replicates is shown, and is representative of two independent experiments. ( d ) Phase-contrast and OCT4, Brachyury and GATA4 immunofluorescence images of cells treated with Wnt3a for 7 days in standard hESC media, N2B27 or mTeSR1. Scale bar, 200 μm. ( e ) Phase-contrast images of hESCs treated for 4 days with Wnt3a in N2B27 media alone, or the same supplemented with 20% PBS or 20% knockout serum replacement (KOSR). Scale bar, 200 μm. ( f ) AP staining of hESC treated for 3 days with Wnt3a in standard hESC media, or the same media in which the KOSR concentration was reduced to 2%. Scale bar, 200 μm. ( g ) Phase contrast and GFP fluorescence in live colonies after 5 days of growth on N2B27 in the presence of vehicle, 20% PBS or 20% KOSR. Scale bar, 200 μm. ( h , i ) Gene expression analysis in cells grown in N2B27 plus the indicated combination of vehicle, Wnt3a and KOSR for four passages. Values were normalized to glyceraldehyde 3-phosphate dehydrogenase, and are expressed relative to vehicle-treated cells at passage 1. The average and range of two biological replicates is shown. Full size image Influence of lysophosphatidic acid (LPA) in serum replacement medium To identify the factor(s) responsible for conferring different Wnt signalling activities in various media, we screened for components of standard hESC medium that could prevent Wnt-mediated differentiation in defined conditions. We found that adding knockout serum replacement (KOSR) to N2B27 or mTeSR1 media efficiently blocked the Wnt-mediated differentiation ( Fig. 3e and Supplementary Fig. S3A ). Conversely, reducing the concentration of KOSR in standard hESC conditions from 20 to 2% allowed Wnt3a-mediated differentiation ( Fig. 3f ), showing KOSR was the key difference between culture systems. In agreement, KOSR addition to N2B27 allowed expansion of hESCs colonies in the presence of Wnt3a for three passages ( Supplementary Fig. S3B ), it prevented loss of OCT4 protein expression on Wnt addition to either N2B27 ( Supplementary Fig. S3C ) or mTeSR1 media ( Supplementary Fig. S3D ), and it prevented the gene expression changes associated with Wnt3a-mediated differentiation on N2B27 media ( Fig. 3h ). Importantly, KOSR did not affect the ability of Wnt3a to activate the TCF-GFP reporter ( Fig. 3g and Supplementary Fig. S3C,D ), showing that KOSR did not interfere with Wnt signal transduction, rather KOSR blocked the loss of pluripotency otherwise caused by Wnt signalling in defined media. Even though hESCs treated with Wnt plus KOSR exhibited pluripotency, they also expressed elevated levels of Brachyury and Mixl1 mRNA, two well-established markers of primitive streak cells ( Fig. 3i ). Co-staining of OCT4 and Brachyury showed that Brachyury was broadly upregulated throughout the OCT4-positive cells in Wnt3a-treated colonies ( Supplementary Fig. S4 ). Furthermore, the co-expression of primitive streak markers and pluripotency markers in Wnt3a-treated hESCs was not due to slow or delayed differentiation as these cells could be expanded for more than ten passages in the presence of Wnt3a and KOSR, maintaining high expression of pluripotency markers indefinitely ( Supplementary Fig. S5A–D ). Likewise, hESCs treated with IWP2 could also be expanded for more than ten passages while retaining equally high levels of pluripotency markers and reduction of primitive streak markers. Therefore, in the presence of KOSR, Wnt signalling does not significantly enhance or reduce expression of pluripotency markers, but it does induce expression of primitive streak markers in undifferentiated cells. KOSR is a partially defined supplement used to replace serum in a variety of cell culture applications. To determine which component(s) of KOSR were responsible for blocking hESC differentiation, we separated the ingredients of KOSR by size using a series of molecular-weight cutoff filters. We tested each fraction for the ability to prevent Wnt-mediated morphological changes. The active component was found to reside in the 50–100 kDa fraction ( Fig. 4a ). The only ingredient in this fraction that was not also found in either N2B27 or mTeSR1 media was a lipid-rich BSA supplement called AlbuMaxII. AlbuMaxII is present at about 1.6% (w/v) in standard hESC culture conditions, and was able to fully substitute for KOSR at this concentration ( Fig. 4b ). As BSA is already present in N2B27 at 500 μg ml −1 , and further supplementation with lipid-free BSA up to 1 mg ml −1 was not able to substitute for AlbuMaxII, we suspected that the active ingredient was one of the lipids associated with BSA. LPA is one of the lipids known to be associated with BSA in serum, and has been implicated in hESC biology previously [17] . Indeed, we found that 10 μM LPA could substitute for 20% KOSR in preventing Wnt3a-mediated differentiation hESCs in defined conditions ( Fig. 4b ). As with KOSR, neither AlbuMaxII nor LPA affected the ability of Wnt3a to activate Wnt signalling in hESCs ( Fig. 4b,c ). 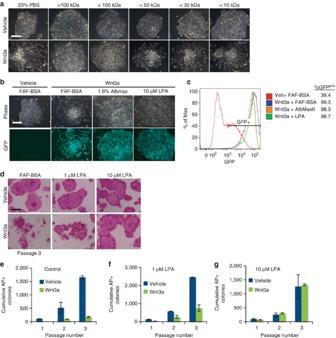Figure 4: Lysophosphatidic acid (LPA) accounts for much of KOSR activity in blocking Wnt-mediated differentiation. (a) KOSR was filtered through different molecular-weight cutoff (MWCO) filters. The flow-through containing proteins smaller than the MWCO at their original concentration was added to 20% (v/v) in N2B27 media. The ability of Wnt3a to induce morphological changes after 3 days was used to determine which fraction contained the factor(s) that prevent Wnt-mediated differentiation. The >100 kDa is enriched for this size, but still contains all smaller proteins at ¼ of the original concentration. Phase-contrast images of hESCs on N2B27 treated with vehicle (Veh) or Wnt3a plus the indicated fraction of KOSR for 3 days are shown. Scale bar, 200 μm. (b) TCF-GFP hESCs were grown on N2B27 plus 20% PBS, 1.5% fatty acid-free BSA (FAF-BSA), 1.6% AlbuMaxII (Invitrogen) or 10 μM LPA supplemented with 1% BSA. Phase-contrast and GFP fluorescence images are shown for cells treated with Veh or Wnt3a for 3 days. Scale bar, 200 μm. (c) FACS analysis of cells inbshowing the fraction of WnthighhESCs. (d) hESCs were grown in N2B27 media, except that irradiated feeders were usedin lieuof Matrigel, for three passages in the presence of 1% FAF-BSA, 1 μM LPA or 10 μM LPA. Veh or Wnt3a was added fresh daily throughout. Alkaline phosphatase (AP) staining after three passages is shown. Scale bar, 500 μm. (e–g) The cumulative number of AP-positive colonies present after each of three passages in the indicated conditions are shown. The average ±s.d. of three biological replicates is shown. Figure 4: Lysophosphatidic acid (LPA) accounts for much of KOSR activity in blocking Wnt-mediated differentiation. ( a ) KOSR was filtered through different molecular-weight cutoff (MWCO) filters. The flow-through containing proteins smaller than the MWCO at their original concentration was added to 20% (v/v) in N2B27 media. The ability of Wnt3a to induce morphological changes after 3 days was used to determine which fraction contained the factor(s) that prevent Wnt-mediated differentiation. The >100 kDa is enriched for this size, but still contains all smaller proteins at ¼ of the original concentration. Phase-contrast images of hESCs on N2B27 treated with vehicle (Veh) or Wnt3a plus the indicated fraction of KOSR for 3 days are shown. Scale bar, 200 μm. ( b ) TCF-GFP hESCs were grown on N2B27 plus 20% PBS, 1.5% fatty acid-free BSA (FAF-BSA), 1.6% AlbuMaxII (Invitrogen) or 10 μM LPA supplemented with 1% BSA. Phase-contrast and GFP fluorescence images are shown for cells treated with Veh or Wnt3a for 3 days. Scale bar, 200 μm. ( c ) FACS analysis of cells in b showing the fraction of Wnt high hESCs. ( d ) hESCs were grown in N2B27 media, except that irradiated feeders were used in lieu of Matrigel, for three passages in the presence of 1% FAF-BSA, 1 μM LPA or 10 μM LPA. Veh or Wnt3a was added fresh daily throughout. Alkaline phosphatase (AP) staining after three passages is shown. Scale bar, 500 μm. ( e – g ) The cumulative number of AP-positive colonies present after each of three passages in the indicated conditions are shown. The average ±s.d. of three biological replicates is shown. Full size image Despite the ability of LPA to block Wnt-mediated differentiation in hESCs, we could not maintain undifferentiated hESCs on defined media (N2B27 media+Matrigel) in the presence of LPA for more than two or three passages, regardless of whether Wnt3a was present or not. However, hESCs could also be expanded in N2B27 media when mouse embryonic fibroblast (MEF) feeders cells were used in lieu of Matrigel, and we found that Wnt3a also induced differentiation of hESCs under these conditions, albeit slower than in media lacking feeders ( Fig. 4d compare with Fig. 3a ). Addition of either 1 or 10 μM LPA resulted in a dose-dependent block in Wnt3a-mediated differentiation, allowing normal expansion of AP+ hESCs in the presence of Wnt3a for three passages ( Fig. 4e–g ). LPA is a lipid-signalling molecule with known roles in early development (for review see refs 17 , 18 , 19 , 20 ) It is known to signal through at least seven different G-protein-coupled receptors. We found that Ki16425, an inhibitor of signalling through LPA receptors 1 and 2 (ref. 21 ), did not abrogate the affects of LPA, suggesting hESCs use one of the other receptors. Taken together, these data uncover a role for lipids in hESC biology. Differentiation of Wnt high and Wnt low cells During gastrulation, cells that enter the primitive streak form the mesodermal and endodermal germ layers, whereas neuroectodermal cells are formed from cells outside the primitive streak [22] . Wnt signalling is highly active in the primitive streak [23] , [24] , [25] , therefore, we asked whether the level of Wnt signalling in undifferentiated hESCs would affect their differentiation potential when self-renewal conditions were removed. The lower expression of primitive streak markers in the Wnt low TCF-GFP hESCs ( Fig. 1d ) and in IWP2-treated non-transgenic hESCs ( Supplementary Fig. S6 ) suggested that these cells had neuroectodermal potential. We directed the differentiation of hESC towards the neural lineage by omitting FGF2 and adding Noggin and SB431542 (ref. 26 ). IWP2-treated cells formed more Pax6+ and Otx2+ neuroectodermal cells than untreated hESCs or Wnt3a-treated hESCs ( Fig. 5a,b ). In fact, hESCs maintained on N2B27 plus Wnt3a and KOSR did not form a single Pax6-positive cell in this assay, indicating that Wnt3a imparts a very strong block in neuroectodermal differentiation in vitro . Consistently, when TCF-GFP hESCs grown in standard hESC conditions were sorted into Wnt low and Wnt high populations and subjected to the neural differentiation protocol, Wnt low cells formed more than 25-fold more Pax6+ neuroectodermal cells than Wnt high cells ( Fig. 5c ). These data suggest a model in which elevated Wnt signalling in the presence of KOSR traps hESCs in a primitive streak-like state from which they cannot differentiate into neuroectodermal cells. 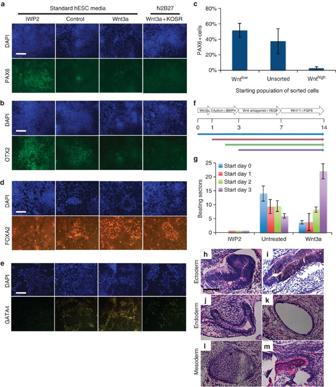Figure 5: Distinct lineage-specific differentiation propensities of Wntlowand WnthighhESCs. (a,b) hESCs maintained with various levels of Wnt pathway activation were subjected to the neural differentiation protocol for 5 days. Neuralectodermal differentiation was detected by immunostaining for Pax6 (a) and Otx2 (b). Scale bar, 200 μm. (c) FACS-sorted populations of >95% pure TCF-GFPhighor TCF-GFPlowwere subjected to the neural differentiation protocol for 5 days. Neural differentiation was detected by PAX6 staining, and compared with the number of DAPI-positive nuclei using an automated counting algorithm. Average ±s.d. from five fields of view, representing three independent experiments. (d) Immunofluorescent staining for endodermal marker FoxA2 in hESCs subjected to the neural differentiation protocol for 5 days. Scale bar, 200 μm. (e) Immunofluorescent staining for endodermal marker Gata4 on day 5 of the endodermal differentiation protocol. Scale bar, 200 μm. (f) Schematic description of cardiogenic differentiation protocol. (g) IWP2- and Wnt3a-treated hESCs in standard hESC media were subjected to the cardiogenic differentiation protocol, and shortened versions thereof. The number of spontaneously beating sectors observed on days 15–18 of the full-length protocol (days 12–15 of the shortest protocol) were averaged. Error bars ±s.d.,n=4. (h–m) Hematoxylin and eosin staining of tumours arising 8 weeks after injecting hESCs maintained in N2B27 with Wnt3a and KOSR for five passages under the kidney capsule of nude mice. (h) Neural rosette, (i) pigmented epithelium, (j,k) glandular structures, (l) cartilage and (m) bone. Scale bar, 50 μm. Figure 5: Distinct lineage-specific differentiation propensities of Wnt low and Wnt high hESCs. ( a , b ) hESCs maintained with various levels of Wnt pathway activation were subjected to the neural differentiation protocol for 5 days. Neuralectodermal differentiation was detected by immunostaining for Pax6 ( a ) and Otx2 ( b ). Scale bar, 200 μm. ( c ) FACS-sorted populations of >95% pure TCF-GFP high or TCF-GFP low were subjected to the neural differentiation protocol for 5 days. Neural differentiation was detected by PAX6 staining, and compared with the number of DAPI-positive nuclei using an automated counting algorithm. Average ±s.d. from five fields of view, representing three independent experiments. ( d ) Immunofluorescent staining for endodermal marker FoxA2 in hESCs subjected to the neural differentiation protocol for 5 days. Scale bar, 200 μm. ( e ) Immunofluorescent staining for endodermal marker Gata4 on day 5 of the endodermal differentiation protocol. Scale bar, 200 μm. ( f ) Schematic description of cardiogenic differentiation protocol. ( g ) IWP2- and Wnt3a-treated hESCs in standard hESC media were subjected to the cardiogenic differentiation protocol, and shortened versions thereof. The number of spontaneously beating sectors observed on days 15–18 of the full-length protocol (days 12–15 of the shortest protocol) were averaged. Error bars ±s.d., n =4. ( h – m ) Hematoxylin and eosin staining of tumours arising 8 weeks after injecting hESCs maintained in N2B27 with Wnt3a and KOSR for five passages under the kidney capsule of nude mice. ( h ) Neural rosette, ( i ) pigmented epithelium, ( j , k ) glandular structures, ( l ) cartilage and ( m ) bone. Scale bar, 50 μm. Full size image If Wnt signalling confers primitive streak characteristics to hESCs, then Wnt high cells should have an advantage in endodermal and mesodermal differentiation. Indeed, Wnt3a-treated hESCs differentiated into endodermal cells far more efficiently than IWP2-treated hESCs in two different assays. First, instead of forming neuroectodermal cells on addition of Noggin and SB431542, Wnt3a-treated cells readily formed FOXA2-positive endodermal cells ( Fig. 5d ), whereas IWP2-treated cells did not. Second, when BMP4 and Activin A were used to direct differentiation towards primitive streak derivatives [27] , Wnt3a-treated hESCs formed more GATA4+ cells with higher average GATA4 expression than either the untreated or IWP2-treated hESCs ( Fig. 5e ). IWP2-treated hESCs formed few GATA4+ cells, all of which had lower average GATA4 expression than the other populations. These data demonstrate the enhanced endodermal differentiation propensity of Wnt high hESCs. In addition, we tested for mesodermal differentiation potential by comparing the ability of IWP2- or Wnt3a-treated hESCs to differentiate into beating cardiomyocytes. We used a four-stage protocol [28] in which pluripotent hESCs are induced to form beating cardiomyoctes over the course of 2 weeks ( Fig. 5f ). We subjected IWP2-treated, Wnt3a-treated and untreated hESCs to the full protocol, as well as a series of shortened protocols to determine whether starting with Wnt high cells could shorten the time it takes to derive cardiomyocytes. Cardiac differentiation was scored by counting the number of beating sectors present on day 15 of the full-length protocol. When starting from untreated hESCs, we found that the full-length protocol resulted in the highest number of beating sectors, as expected ( Fig. 5g ). Wnt3a-treated hESCs on the other hand formed the most beating sectors when the first two stages of differentiation were eliminated entirely. In fact, Wnt3a-treated hESCs subjected to only the last two stages of differentiation formed more beating sectors than untreated hESCs given the full-length protocol. Thus, using Wnt3a and KOSR to maintain hESCs resulted in faster, more efficient-directed differentiation into cardiomyocytes and endodermal cells. Wnt low hESCs formed few beating sectors regardless of protocol length, consistent with their neuroectodermal-specific differentiation propensity. Therefore, by including IWP2 or Wnt3a+KOSR in the self-renewal medium, hESCs can be expanded indefinitely in a state that allows faster and more efficient differentiation towards neuroectodermal or mesodermal/endodermal cell types, respectively. Finally, given the strong differentiation biases of Wnt low and Wnt high hESCs, we questioned whether these cells were still pluripotent. Strong expression of pluripotency markers in both populations ( Supplementary Fig. S5A–D ) suggested this was the case, but teratoma formation is the best measure of pluripotency in hESCs. Therefore, we injected Wnt high hESCs under the kidney capsule of nude mice and examined the resulting tumours 8 weeks later. We found evidence of differentiation into all three germ layers in every tumour ( Fig. 5h–m ), showing these cells remained pluripotent even after five passages in the presence of Wnt3a and KOSR media. In agreement, removal of Wnt3a or IWP2 from any culture resulted in re-establishment of heterogeneous TCF-GFP expression levels within three passages. Thus, both the level of Wnt signalling ( Fig. 1e,f ) and the lineage-specific differentiation biases of hESCs ( Fig. 5h–m ) are reversible phenotypes. In hESCs cultured under standard conditions, this reversibility leads to a dynamic equilibrium of individual hESCs with distinct differentiation biases, thereby limiting the efficiency with which any single lineage can be targeted. Our data show that different levels of Wnt signalling confer distinct lineage-specific differentiation propensities to hESCs. Wnt low /IWP-treated cells are maintained as pluripotent cells, and show enhanced ability to differentiate into neural cells on inhibition of transforming growth factor-β signalling. Wnt-treated hESCs, on the other hand, acquire primitive streak-like characteristics and, in defined self-renewal media, rapidly differentiate into mesodermal and endodermal cells. In the presence of KOSR, however, Wnt still drives hESCs towards a primitive streak-like state, but differentiation is blocked before loss of pluripotency. hESCs in this fluid pluripotent/primitive streak-like state can be expanded indefinitely, and can differentiate into mesodermal and endodermal cells with greater speed and efficiency than heterogeneous populations. The ability of KOSR to block Wnt-mediated loss of pluripotency and enhance clonogenicity reconciles many of the discrepancies among reports using different self-renewal media to assess the role of Wnt signalling in hESCs [7] , [8] , [9] , [10] , [11] , [12] , [13] . Further discrepancies have arisen from the fact that Wnt signalling simultaneously increases self-renewal ( Fig. 3a,b ) and traditional markers of differentiation ( Fig. 3i ) when added to hESCs in the presence of KOSR. Finally, it is worth noting that the role for Wnt3a in hESCs identified herein is significantly different from the role that we and others have shown for Wnt3a in mouse ESCs [14] , [29] , [30] , [31] . In the latter case, Wnt3a blocked developmental progression from the naive mESC state [14] to the primed EpiSC state; whereas the primary role of Wnt in hESCs is to drive differentiation out of the pluripotent primed state of hESCs and into differentiated mesodermal and endodermal cells. Cell culture Routine culture of H9 hESCs was performed on a feeder layer of irradiated CF1α MEFs at 20,000 cells per cm 2 in 'standard hESC media' (DMEM/F12, 20% KOSR (Invitrogen), 10 ng ml −1 basicFGF (Peprotech), 1% MEM non-essential amino acids, 0.1 mM β-mercaptoethanol and 1 mM glutamine). Cells were passed as clumps following 30 min digestion with 1 mg ml −1 collagenase IV, every 4–6 days. Cells cultured in N2B27-CDM [14] or mTeSR1 (Stemcell Technologies) were grown on Matrigel (BD Biosciences)-coated tissue culture plastic instead of MEFs, and passed as clumps using 1 mg ml −1 dispase instead of collagenase IV. Recombinant mouse Wnt3a was produced in Drosophila S2 cells grown in suspension culture, and purified by affinity and gel filtration chromatography as described [32] . Wnt3a protein was used at 100 μg ml −1 , IWP2 (Stemgent) at 2 μM, and CHIR99021 (Stemgent) at 3 μM. All reagents were changed daily in all experiments herein, except during the cardiac differentiation protocol. Generation of transgenic Wnt reporter hESCs Three independent monoclonal transgenic Wnt reporter lines were generated by transducing three separate pools of hESCs with a lentivirus harbouring a 7xTCF-eGFP construct and puromycin resistance gene [14] . Transduced pools were selected with puromycin 4 days after transduction, cultured separately for 2 weeks to allow viral silencing to proceed and then plated as single cells in standard hESC conditions in the presence of ROCK inhibitor Y27632 (ref. 33 ) to allow clonal outgrowth. After 5 days of clonal outgrowth, Wnt3a was added for 24 h and one Wnt-responsive colony from each pool was selected for expansion and experimentation. Quantitative clonogenic potential assay hESCs were digested to single cells using Accutase, FACS sorted in some cases, counted and plated at 500–2,500 cells per cm 2 in 'standard hESC media' [1] , [2] . AP activity was detected 7 days later using the SCR004 kit (Millipore). In some cases, colonies were fixed and stained for OCT4 to get an independent measurement of clonogenic potential. For experiments using multiple passages, duplicate wells were grown, one of which was used for clonogenic potential assay, the other being used for passage. AP+ colonies were counted by hand using a dissecting microscope. These experiments were performed in duplicate (TCF-GFP high versus TCF-GFP low ), triplicate (Wnt3a and CHIR99021 on all media) or quadruplicate (IWP2 on all media). Directed differentiation protocols Differentiation of hESC towards endoderm was accomplished using stage one of the protocol described in ref. 27 . hESC were treated with Y-27632 for 1 h before digesting to single cells using Accutase (Stemgent). Single cells were plated at 50,000 cells per cm 2 in N2B27 media supplemented with 10 μM Y-27632. Twenty-four hours later, media were changed to StemPro-34 (Invitrogen), 2 mM glutamine, 0.4 mM monothioglycerol, 50 μg ml −1 ascorbic acid, 3 ng ml −1 Activin A (R&D Systems), 10 ng ml −1 BMP4 (R&D Systems) and 5 ng ml −1 FGF2 (Peprotech). Differentiating cells were fixed and stained for 4',6-diamidino-2-phenylindole (DAPI) and GATA4 after 4 days of differentiation. Differentiation of hESC towards neuroectoderm used the protocol described in ref. 26 . Briefly, hESCs pretreated with Y-27632 for 1 h were digested to single cells with Accutase. Single cells were plated at 60,000 cells per cm 2 in N2B27 media supplemented with 10 μM Y-27632. Twenty-four hours later, media was changed to SN media (similar to standard hESC media, except lacking FGF2 and containing with 50 ng ml −1 human recombinant Noggin (R&D Systems) and 10 μM SB431542 (Stemgent)). Cells were fixed and stained for DAPI, Pax6, Otx2 and FoxA2 after 5 days in SN media. Cardiogenic differentiation was induced following the protocol reported in refs 27 , 28 . Approximately 1×10 6 hESCs of each population were digested into clumps of 100–200 cells using collagenase IV and slight trituration. hESC clumps were washed and resuspended in mTeSR1 media, and plated at 200,000 cells per well in ultra-low-adherence six-well plates. Cardiovascular differentiation was initiated the following day (day 0) by changing the base media to StemPro-34 supplemented with 2 mM glutamine, 0.4 mM monothioglycerol and 50 μg ml −1 ascorbic acid. The base media was supplemented with the cytokines: 50 ng ml −1 Wnt3a for day 0–1; 20 ng ml −1 each BMP4, VEGF and Activin A for days 1–3; 50 ng ml −1 soluble Frizzled-8 CRD [34] plus 10 ng ml −1 VEGF for days 3–5; 50 ng ml −1 each FGF8 and Wnt11 for days 5–9, 9–13 and 13–17. To determine whether Wnt high hESCs had any cardiovascular differentiation advantages, separate pools of hESC aggregates were subjected to this protocol beginning on Day 0, 1, 2 or 3. Beating sectors were counted in each condition on protocol days 14–16 and averaged. Immunohistochemistry Cells were fixed in 4% paraformaldehyde for 15 min, washed twice with PBS/0.5% Triton X-100 (PBT), permeabilized for 10 min with 0.1% Tween-20 in PBS, and blocked with 5% normal donkey serum or 10% BSA for 1 h. Cells were incubated with primary antibody (see below) diluted in blocking buffer overnight at 4 °C, washed three times with PBT, incubated with species-specific secondary antibodies conjugated to Alexa488 or Cy3 for 1 h at room temperature (Jackson ImmunoResearch), washed three times with PBT, and imaged on an Axiovert 200 inverted microscope with an Axiocam HRc camera (Carl Zeiss). Images were analysed using AxioVision 4.8.2 software (Zeiss). Fluorescence-activated cell sorting hESC colonies were dissociated to single cells with Accutase, pelleted and resuspended in PBS/10% serum for staining with antibodies (see below). Rat anti-mouse CD29-APC (BioLegend, 1:200) was used identify and exclude mouse feeder cells, propidium iodide (3 μg ml −1 ) was used to identify and exclude dead cells. Cells were analysed and sorted on a FACSAria II cell sorter (BD Biosciences). FACS data were analysed with the FlowJo software (TreeStar). GFP gates were set based on differences in the GFP expression profile of IWP2-Wnt3a-treated hESCs, other gates were set based on florescence minus one control samples, which lacked the primary antibody of interest, but contained all other antibodies and stains. For clonogenic and GFP reversion analyses, cells were pretreated with 10 μM Y-27632 for 1 h before digestion. Cell proliferation was measured using the Click-iT Edu Cell Proliferation Assay for Flow Cytometry (Invitrogen). hESCs in log-phase growth were pulsed with Edu for 3 h before processing. Data are shown only for OCT4-positive cells for two reasons: to avoid obscuring the role of Wnt in undifferentiated cells by including differentiating cells in the analysis and to allow elimination of mouse feeder cells from the analysis without needing to stain for CD29. Antibodies and flow cytometry Antibodies were used at the following concentrations: Oct4 (Santa Cruz Biotechnology, 1:100), Nanog-PE (BD Pharmingen, 1 test per ml), SSEA3-Alexa488 (eBiosciences, 1 test per ml), SSEA4-PE (R&D Systems, 0.5 test per ml), TRA160-FITC (Biolegend, 1:100), Pax6 (Covance, 1:2,000), Otx2 (Abcam, 1:2,000), FoxA2/HNF3β (Santa Cruz Biotechnology, 1:250), GATA4-Biotin (R&D Systems, 1:50), Brachyury-Bio (R&D Systems, 1:50) and GFP (Abcam, 1:1,000). Gene expression analysis Total RNA was prepared using a QIAGEN RNeasy mini kit with on-column DNase digestion, followed by random hexamer-primed reverse transcription using Superscript III RT-PCR kit (Invitrogen). Quantitative real-time PCR was performed on a StepOne Plus (Applied Biosystems) using a SYBR green technology. Standard curves were performed for each gene in every run, and all PCR reactions were performed for three independent experiments with two technical replicates in each experiment. Glyceraldehyde 3-phosphate dehydrogenase was used to normalize all samples for starting material. Primer sequences were designed using Lightcycler Probe Design Software 2.0 (Roche) such that they spanned splice junctions when possible ( Supplementary Table S1 ). Kidney capsule transplantation and teratoma analysis A total of 1×10 6 hESCs maintained in NWKI media (N2B27 media plus 100 μg ml −1 Wnt3a, 20% KOSR and 2 μM IWP2) for five passages were mixed with Matrigel (BD Biosciences) at 1:1 ratio and transplanted under the kidney capsule of SCID mice. Transplanted kidney capsules were collected after 6–8 weeks, fixed in 4% PFA, embedded in paraffin, cut to 5 μM section on a microtome and stained with hematoxylin and eosin. All procedures were conducted in accordance with the Stanford Administrative Panel for Laboratory Animal Care guidelines. How to cite this article: Blauwkamp, T.A. et al . Endogenous Wnt signalling in human embryonic stem cells generates an equilibrium of distinct lineage-specified progenitors. Nat. Commun. 3:1070 doi: 10.1038/ncomms2064 (2012).